Deletion of cavin genes reveals tissue-specific mechanisms for morphogenesis of endothelial caveolae Caveolae are abundant in endothelial cells and are thought to have important roles in endothelial cell biology. The cavin proteins are key components of caveolae, and are expressed at varied amounts in different tissues. Here we use knockout mice to determine the roles of cavins 2 and 3 in caveolar morphogenesis in vivo . Deletion of cavin 2 causes loss of endothelial caveolae in lung and adipose tissue, but has no effect on the abundance of endothelial caveolae in heart and other tissues. Changes in the morphology of endothelium in cavin 2 null mice correlate with changes in caveolar abundance. Cavin 3 is not required for making caveolae in the tissues examined. Cavin 2 determines the size of cavin complexes, and acts to shape caveolae. Cavin 1, however, is essential for normal oligomerization of caveolin 1. Our data reveal that endothelial caveolae are heterogeneous, and identify cavin 2 as a determinant of this heterogeneity. Caveolae have a range of functions, playing important roles in adipocyte metabolism and lipid homoeostasis, in cellular mechanosensation, and in endothelial cell biology, as well as other processes [1] , [2] , [3] , [4] . Caveolae comprise around 20% of the surface of continuous microvascular endothelium [5] , [6] , [7] , and are linked to endothelial permeability by several different observations. Electron microscopy suggests that budding of caveolae from one side of the endothelial cell and fusion at the other side may constitute a mechanism for endothelial transcytosis [8] , [9] , [10] . Imaging of antibodies against caveolar proteins reveals that these antibodies are efficiently pumped from blood to surrounding tissue [11] . Endothelial pores share common protein components with caveolae, particularly the protein PV-1 (refs 12 , 13 , 14 ). Further experiments reveal a role for caveolae in the regulation of endothelial nitric oxide synthase signalling, which impacts directly on the permeability state of endothelial paracellular junctions [3] , [15] , [16] . The molecular cell biology underlying these processes remains largely unknown. Recent research has identified a protein family, the cavins, which are crucial for the formation of caveolae [17] , [18] , [19] , [20] , [21] , [22] , [23] . Previously, the only proteins established in this process were the caveolins. There are three caveolins in mammals. Caveolins 1 and 2 are abundant in endothelium and adipose tissue, and are expressed at lower levels in other tissues excluding striated muscle. Caveolin 3 is restricted to striated muscle [24] . Intriguingly, caveolin 1 alone can generate caveolae-like membrane vesicles in a completely heterologous system [25] , so it is likely that the expression of the cavins provides additional functional and regulatory complexity. There are four cavins in mammals. Cavins 1 to 3 are widely expressed, while cavin 4 is, like caveolin 3, expressed only in striated muscle [26] . In this paper we use the cavin names, but it should be noted that these are not the standard gene names for this family ( cavin 1 = Ptrf , cavin 2 = Sdpr , cavin 3 = Prkcdbp , cavin 4 = Murc . Cavin 3 is also frequently referred to as SRBC [17] ). The cavin proteins form hetero-oligomeric complexes [18] , [27] . They are expressed at different abundances in various tissues, leading to the hypothesis that the presence of different complements of cavin proteins could generate differences between caveolae in diverse tissues or cell types [17] , [27] . Direct evidence to support this hypothesis has been lacking. Knockout mice for the caveolin 1 or cavin 1 genes have been generated previously [28] , [29] , [30] , [31] , and display a similar range of complex lipodistrophic and other metabolic defects that may be linked to the role of caveolae in adipocytes [1] , [28] , [32] , [33] . Endothelial barrier function and other cardiovascular parameters have yet to be fully analysed in the cavin 1 −/− mice, but there are several reports that endothelial permeability to albumin is increased in caveolin 1 −/− mice [3] , [9] , [34] , [35] , [36] . This implies that, if caveolae do indeed mediate endothelial transcytosis, compensatory mechanisms must exist to actually increase albumin efflux from blood vessels in their absence. In agreement with this, there is evidence for opening of endothelial tight junctions in the lung of caveolin 1 −/− mice [3] , [34] , [36] . In this paper, we report the generation of cavin 2 −/− and cavin 3 −/− mice, and analyse cells and tissues from these mice alongside those from caveolin 1 −/− and cavin 1 −/− strains. We have used biochemical, imaging and electron microscopy methods to study the requirements for different cavins in the formation of morphologically defined caveolae in the endothelium of different tissues, and in cultured endothelial cells. We have also used complementary approaches to assess alterations in endothelial ultrastructure in the knockout mice. We found that cavin 3 does not appear to be needed for generating endothelial caveolae, and the morphology of the endothelium in cavin 3 −/− mice is normal. Cavin 2 , however, has an important role specifically in generating caveolae in lung and fat endothelia. The apparent size of the protein complexes into which cavins assemble is smaller in the lung and fat compared with other tissues. Cavin 2 is responsible for determining the size or stability of cavin complexes, as deletion of cavin 2 actually increases the apparent size of cavin complexes in the lung. In both the endothelium of the lung and in cultured lung endothelial cells, the residual caveolae detected in the absence of cavin 2 have a reduced depth. Moreover, in cavin 2 −/− cells other caveolar components such as cavin 1 and caveolin 1 are detected in flat regions of the plasma membrane and shallow caveolae. We conclude that endothelial caveolae in different tissues are heterogeneous, that cavin 2 has an important role in generating such heterogeneity, and that the role of cavin 2 in caveolar morphogenesis is directly linked to determining the membrane shape of caveolae. Generation of cavins 2 −/− and 3 −/− mice We imported mice lacking caveolin 1 (ref. 30 ), and backcrossed them for seven generations onto the strain C57Bl/6. We imported mice lacking cavin 1 , already on the C57Bl/6 background [28] . We generated mice lacking cavin 2 and mice lacking cavin 3 , using C57Bl/6 embryonic stem cells ( Supplementary Fig. S1 ), and following germ-line transmission of the null mutation backcrossed these onto C57Bl/6 for four generations. As one would predict given the previous characterization of caveolin 1 −/− and cavin 1 −/− mice, all four null strains were viable and fertile with no gross phenotypes [28] , [30] , [31] , [37] . However, in crosses where both parents were heterozygous for cavin 1 there was a significant deviation from the predicted frequency of homozygous knockout pups (In heterozygous x heterozygous crosses percentage of homozygous knockout pups at weaning was 26% for cavin 2 ( N =195), 29% for cavin 3 ( N =235), 13% for cavin 1 ( N =137) and 25% for caveolin 1 ( N =106)). Western blotting of a range of tissues from the knockout mice and congenic controls confirmed that the caveolin 1, cavin 1, cavin 2 and cavin 3 proteins are indeed absent in the relevant strains ( Fig. 1 and Supplementary Fig. S2 ). Changes in cavin 1 and caveolin 2 expression in caveolin 1 −/− mice and caveolin 1 and 2 expression in cavin 1 −/− mice were consistent with previous reports [20] , [27] , [38] . Deletion of cavin 1 caused loss of cavin 2 and 3 proteins, but cavin 2 −/− and cavin 3 −/− mice had unaltered levels of cavin 1 and caveolin 1 ( Fig. 1 ). Similarly, cavin 2 levels were not altered when cavin 3 was deleted. However, there was consistent upregulation of cavin 3 in cavin 2 −/− mice across all tissues examined. This was the case even in tissues, such as kidney, spleen, testis, brain and muscle, where cavin 2 could not be detected by western blotting ( Fig. 1 and Supplementary Fig. S2 ). These data from western blotting of tissues from the different knockout mice show that cavins 2 and 3 are not stably expressed in the absence of cavin 1 or caveolin 1 , confirm that the ratio between the different cavins is markedly different in different tissues [27] and demonstrate that deletion of cavin 2 or cavin 3 does not reduce the levels of other caveolar proteins. In addition, western blotting with antibodies against the recently identified caveolar protein EHD2 (refs 23 , 39 , 40 , 41 ) showed that this protein is also expressed at reduced levels in caveolin 1 −/− and cavin 1 −/− mice, thereby providing direct evidence that it is likely to be linked to caveolar function in vivo . 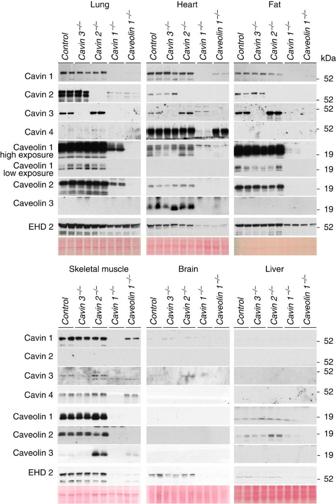Figure 1: Protein expression levels incavin 1–3andcaveolin 1knockout mice. Tissues from mice with the indicated genotypes were analysed by western blotting, using antibodies as shown. Note that all samples were obtained and analysed in duplicate. Blots for the lung, heart, fat and liver, and for skeletal muscle and brain, were processed and exposed to film simultaneously, so that the intensity of the bands for each individual protein is meaningfully comparable and gives information on the relative abundance of each protein in the different tissues shown. Ponceau staining of the membranes used for blotting is included to demonstrate equal total protein loading. More tissue types are analysed inSupplementary Fig. S2. Figure 1: Protein expression levels in cavin 1–3 and caveolin 1 knockout mice. Tissues from mice with the indicated genotypes were analysed by western blotting, using antibodies as shown. Note that all samples were obtained and analysed in duplicate. Blots for the lung, heart, fat and liver, and for skeletal muscle and brain, were processed and exposed to film simultaneously, so that the intensity of the bands for each individual protein is meaningfully comparable and gives information on the relative abundance of each protein in the different tissues shown. Ponceau staining of the membranes used for blotting is included to demonstrate equal total protein loading. More tissue types are analysed in Supplementary Fig. S2 . Full size image The different tissue distributions of the cavins could, in principle, reflect either expression in different cell types or changes in relative abundance within the same cell type. In the case of cavin 4 the former is the case, as cavin 4 is expressed predominantly in myocytes of striated muscle [26] , [27] , [42] . In the case of cavin 3 the latter is the case, as cavin 3 and caveolin 1 clearly co-localize in several tissues [19] . The distribution of cavins 1 and 2 within tissues has not been studied in detail. Indirect immunofluorescent labelling of tissue sections with antibodies against cavin 1, cavin 2 and caveolin 1 revealed that in all tissues examined cavin 1, cavin 2 and caveolin 1 co-localize extensively. Cavin 1 and cavin 2 antibodies gave highly specific labelling, as judged using knockout tissue as a negative control ( Supplementary Fig. S3 ). In the heart and in adipose tissue caveolin 1, cavin 1 and cavin 2 are found predominantly in endothelial cells ( Fig. 2 ). In subsequent experiments, we focused on the role of cavins 1, 2 and 3 in generating caveolae in endothelia. 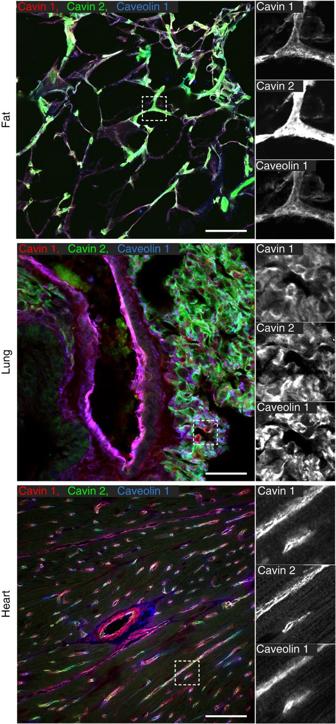Figure 2: Distribution of cavins 1 and 2 in different tissues. Sections of the tissues shown were labelled using indirect immunofluorescence, with antibodies against caveolin 1, cavin 1 and cavin 2. The black and white panels show the areas denoted with a dashed box, the signals from the three antibodies being separated to allow visualization of co-localization. Bars are all 20 μm. Figure 2: Distribution of cavins 1 and 2 in different tissues. Sections of the tissues shown were labelled using indirect immunofluorescence, with antibodies against caveolin 1, cavin 1 and cavin 2. The black and white panels show the areas denoted with a dashed box, the signals from the three antibodies being separated to allow visualization of co-localization. Bars are all 20 μm. Full size image Quantification of the abundance of endothelial caveolae We carried out a survey of the abundance of caveolae in microvascular endothelia in different tissues from control, cavin 1 −/− , cavin 2 −/− , cavin 3 −/− and caveolin 1 −/− mice, aiming to correlate potential changes in caveolar abundance with the differential expression of cavin proteins. Initially, we examined micrographs by eye and scored the abundance of endothelial caveolae using an arbitrary scale ( Supplementary Fig. S4A ). This was done with randomized samples and completely blind to the genotype of each individual sample. This initial study suggested that: (1) caveolae are largely absent in caveolin 1 −/− and cavin 1 −/− tissues, as one would predict [28] , [29] , [30] , [31] ; (2) cavin 3 is not essential for formation of endothelial caveolae in any of the tissues examined; (3) the effects of deletion of cavin 2 are not uniform across endothelia from different tissues, for example, in lung endothelia of cavin 2 −/− mice there were very few structures morphologically identifiable as caveolae, whereas in the heart and muscle, however, there was no noticeable difference between control and cavin 2 −/− mice ( Supplementary Fig. S4A ). As these observations provide direct evidence for different requirements for caveolar morphogenesis in different types of endothelial cell, we sought to confirm them in a quantitative manner. We focused on continuous microvascular endothelium of the lung and the heart. As cavin 3 expression increases in cavin 2 −/− mice ( Fig. 1 , Supplementary Fig. S2 ), we investigated potential functional redundancy or compensatory effects on caveolar abundance between these two cavins by breeding cavin 2 −/− cavin 3 −/− double knockout mice. Multiple electron micrographs were obtained ( Fig. 3a ) and the number of caveolae counted. This was done in control, caveolin 1 −/− , cavin 2 −/− and cavin 3 −/− mice, as well as for cavin 2 −/− cavin 3 −/− double knockouts ( Fig. 3a ). The results confirmed that deletion of cavin 3 does not significantly (using an unpaired t -test) alter the abundance of caveolae. Additionally, cavin 2 is not required for generating caveolae in the heart microvascular endothelia, but in the cavin 2 −/− lung samples the abundance of caveolae in microvascular endothelium was greatly reduced. The abundance of caveolae in the lung and the heart from cavin 2 −/− cavin 3 −/− double knockouts was the same as was observed for cavin 2 −/− samples in both cases, so the differential effects on caveolar abundance in the heart and lung endothelium observed when cavin 2 is deleted are not due to compensatory or functionally redundant processes requiring cavin 3 . 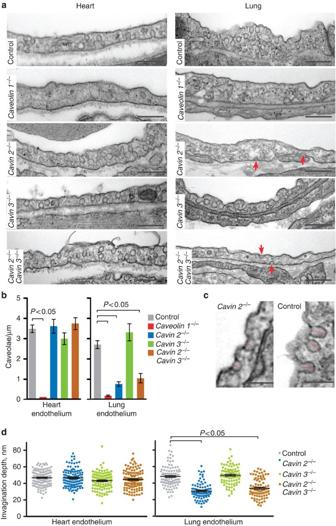Figure 3: Cavin 2 is required for generating endothelial caveolae in lung but not heart. (a)Cavin 2−/−lung endothelium lacks caveolae, butcavin 2−/−heart endothelium has the same abundance of caveolae as congenic controls. Representative electron micrographs are shown, with the relevant genotype indicated. Note the shallow membrane invaginations incavin 2−/−lung andcavin 2−/−cavin 3−/−lung, arrowed. Bars, 500 nm. (b) Quantification of caveolae in the heart and lung microvascular endothelium in tissues from congenic control,caveolin 1−/−,cavin 2−/−,cavin 3−/−, andcavin 2−/−cavin 3−/−mice. Multiple electron micrographs were obtained for each tissue, and both the number of caveolae and total length of plasma membrane present were quantified in each image. Caveolae were counted as omega-shaped membrane profiles open at the cell surface.N>15, bars are s.e.m.,P-values were calculated using an unpairedt-test. (c) Higher-resolution images comparing the depth of membrane invaginations seen incavin 2−/−lung endothelium with caveolae from control lung endothelium. Note that these invaginations are included as morphologically defined caveolae in the quantification shown inb, and are much less frequent than caveolae in control samples, and are not seen incaveolin 1−/−mice. Bars, 100 nm. (d) Quantification of the depth of caveolae in the lung and the heart microvascular endothelium fromcavin 2−/−, cavin 3−/−, andcavin 2−/−cavin 3−/−mice. Depth was measured in electron micrographs from the caveolar opening as illustrated inc.N>100. Figure 3: Cavin 2 is required for generating endothelial caveolae in lung but not heart. ( a ) Cavin 2 −/− lung endothelium lacks caveolae, but cavin 2 −/− heart endothelium has the same abundance of caveolae as congenic controls. Representative electron micrographs are shown, with the relevant genotype indicated. Note the shallow membrane invaginations in cavin 2 −/− lung and cavin 2 −/− cavin 3 −/− lung, arrowed. Bars, 500 nm. ( b ) Quantification of caveolae in the heart and lung microvascular endothelium in tissues from congenic control, caveolin 1 −/− , cavin 2 −/− , cavin 3 −/− , and cavin 2 −/− cavin 3 −/− mice. Multiple electron micrographs were obtained for each tissue, and both the number of caveolae and total length of plasma membrane present were quantified in each image. Caveolae were counted as omega-shaped membrane profiles open at the cell surface. N >15, bars are s.e.m., P- values were calculated using an unpaired t -test. ( c ) Higher-resolution images comparing the depth of membrane invaginations seen in cavin 2 −/− lung endothelium with caveolae from control lung endothelium. Note that these invaginations are included as morphologically defined caveolae in the quantification shown in b , and are much less frequent than caveolae in control samples, and are not seen in caveolin 1 −/− mice. Bars, 100 nm. ( d ) Quantification of the depth of caveolae in the lung and the heart microvascular endothelium from cavin 2 −/− , cavin 3 −/− , and cavin 2 −/− cavin 3 −/− mice. Depth was measured in electron micrographs from the caveolar opening as illustrated in c . N >100. Full size image The residual caveolar membrane invaginations in cavin 2 −/− and cavin 2 −/− cavin 3 −/− lung endothelium frequently appeared more shallow than those observed in control samples ( Fig. 3a ). Morphometric analysis of the depth of these invaginations in cavin 2 −/− and cavin 2 −/− cavin 3 −/− samples confirmed that they are indeed shallower than control caveolae, and revealed that the effect of deleting cavin 2 was the same as deleting both cavin 2 and cavin 3 simultaneously ( Fig. 3d ). Deletion of cavin 2, or deletion of cavin 2 and cavin 3 simultaneously, had no effect on the size or shape of caveolae in the heart endothelium ( Fig. 3d ). The data show, therefore, that cavin 2 is not required for generating caveolae in the heart microvascular endothelium, but that in the microvascular endothelium of lung the deletion of cavin 2 causes a pronounced reduction in the abundance of caveolae. The loss of caveolae in cavin 2 −/− lung is less severe than that observed in caveolin 1 −/− samples, and the shallow caveolar invaginations seen in cavin 2 −/− samples from these tissues are not seen in caveolin 1 −/− samples. This latter observation argues that the invaginations are indeed caveolar in origin, rather than representing a potential separate type of invagination induced by loss of caveolae. The size of cavin complexes varies between tissues Cavin proteins assemble into hetero-oligomeric complexes, and these complexes are likely to be central to cavin function [17] , [27] , [43] . In HeLa cells, cavin complexes can be isolated as a single peak on sucrose velocity gradients following solubilization in 0.5% Triton X100 (ref. 43 ). We applied essentially the same protocol to study the size of cavin complexes in different tissues. The cavins were found in high–molecular-weight complexes, and in all tissues cofractionated with each other ( Fig. 4a (ref. 43 )). However, the fractionation behaviour of cavin complexes was not the same in all tissues examined. In the heart and the kidney, the cavin proteins peaked at a sucrose density of 20–22%. In both lung and fat the cavin complexes had a markedly smaller size, peaking at a sucrose density of 10–12% ( Fig. 4a ). Use of purified 40S and 60S ribosomal subunit as standards indicated that the cavin complexes are a little less than 40S in lung and fat, and around 60S in the other tissues ( Fig. 4c ). These data imply that there are biochemical differences between cavin complexes in different tissues. 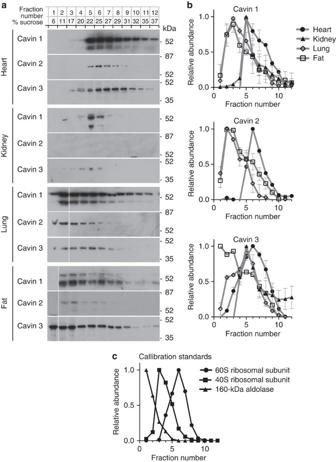Figure 4: Cavin complexes have different apparent sizes in different tissues. (a) Western blots of fractions from sucrose density gradients. Both the fraction number, used for the plots inb, and the experimentally (by refractometer) determined sucrose density from each fraction are shown. Fractions from each tissue (heart, kidney, lung and fat) were probed with antibodies against cavin 1, cavin 2 and cavin 3. (b) Densitometry from western blots as ina, to allow distribution of cavin proteins to be compared in different tissues. Bars represent s.e.m., values are means from three separate experiments. Key indicates which profile is from each tissue. (c) Densitometry from Coomassie blue-stained gels of fractions from velocity gradients of samples containing purified ribosomal subunits, and aldolase, as standards. Figure 4: Cavin complexes have different apparent sizes in different tissues. ( a ) Western blots of fractions from sucrose density gradients. Both the fraction number, used for the plots in b , and the experimentally (by refractometer) determined sucrose density from each fraction are shown. Fractions from each tissue (heart, kidney, lung and fat) were probed with antibodies against cavin 1, cavin 2 and cavin 3. ( b ) Densitometry from western blots as in a , to allow distribution of cavin proteins to be compared in different tissues. Bars represent s.e.m., values are means from three separate experiments. Key indicates which profile is from each tissue. ( c ) Densitometry from Coomassie blue-stained gels of fractions from velocity gradients of samples containing purified ribosomal subunits, and aldolase, as standards. Full size image Lung and fat contain high levels of cavin 2 ( Fig. 1 ). We quantified the abundance of caveolae in cavin 2 −/− adipocytes and cavin 2 −/− endothelium within adipose tissue and found that in both cases there was a loss of caveolae as seen in cavin 2 −/− lung endothelium, while deletion of cavin 3 did not effect caveolar abundance ( Supplementary Fig. S4B ). With these observations in mind, we asked whether the decrease in apparent size of cavin complexes in the lung and fat could be explained by the activity of cavin 2. We carried out sucrose velocity gradient fractionation as for Fig. 4 , analysing the lung and the heart from cavin 2 −/− , cavin 3 −/− and cavin 2 −/− cavin 3 −/− mice, and used western blotting to follow the distribution of cavin 1 on the gradients. In the heart, there was no large change in distribution of cavin 1 in any of the knockout samples, although in the cases of cavin 3 −/− and cavin 2 −/− cavin 3 −/− samples the size of the complexes containing cavin 1 was slightly reduced ( Fig. 5a ). This is what one would predict, as cavins 2 and 3 are likely to be present in those complexes along with cavin 1. In the lung, however, there was a marked increase in the size of cavin 1-containing complexes in cavin 2 −/− samples ( Fig. 4b ), so that the profile of cavin 1 in cavin 2 −/− lungs resembled that observed in control heart. There was a slight decrease in the size of cavin 1 complexes in cavin 3 −/− samples ( Fig. 4b ), and cavin 2 −/− cavin 3 −/− samples contained cavin 1 complexes at increased size relative to controls, but this increase was less pronounced than when cavin 2 alone was absent ( Fig. 4b ). These data imply that cavin 2 has a specific role in controlling the size or stability of cavin complexes, that expression of cavin 2 reduces the size or stability of these complexes and that this activity of cavin 2 may account for the variation in the apparent size of cavin complexes on sucrose gradients observed between the lung and the heart. 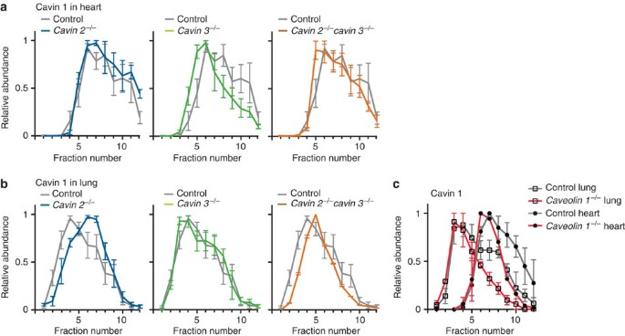Figure 5: Cavin 2 controls the size of cavin complexes. (a) Densitometry from western blots of fractions from sucrose velocity gradients as inFig. 4, comparing the distribution of cavin 1 complexes in the heart from control,cavin 2−/−,cavin 3−/−andcavin 2−/−cavin 3−/−mice. Colour key indicates which profile is from each tissue/genotype. Note that the control data are reproduced in all three panels—values shown are means from three experiments, bars represent s.e.m. (b) Densitometry from western blots of fractions from sucrose velocity gradients as inFig. 4, comparing the distribution of cavin 1 complexes in lung from control,cavin 2−/−,cavin 3−/−andcavin 2−/−cavin 3−/−mice. Colour key indicates which profile is from each tissue/genotype. Note that the control data are reproduced in all three panels—values shown are means from three experiments, bars represent s.e.m. (c) Densitometry from western blots of fractions from sucrose velocity gradients, comparing the distribution of cavin 1 complexes from control andcaveolin 1−/−lung and heart tissues. Colour key indicates which profile is from each genotype. Values shown are means from three experiments, bars represent s.e.m. Note that the absolute abundance of cavin 1 incaveolin 1−/−tissues is much less than controls, and all data are normalized to show relative abundance in different fractions, peak fraction=1. Figure 5: Cavin 2 controls the size of cavin complexes. ( a ) Densitometry from western blots of fractions from sucrose velocity gradients as in Fig. 4 , comparing the distribution of cavin 1 complexes in the heart from control, cavin 2 −/− , cavin 3 −/− and cavin 2 −/− cavin 3 −/− mice. Colour key indicates which profile is from each tissue/genotype. Note that the control data are reproduced in all three panels—values shown are means from three experiments, bars represent s.e.m. ( b ) Densitometry from western blots of fractions from sucrose velocity gradients as in Fig. 4 , comparing the distribution of cavin 1 complexes in lung from control, cavin 2 −/− , cavin 3 −/− and cavin 2 −/− cavin 3 −/− mice. Colour key indicates which profile is from each tissue/genotype. Note that the control data are reproduced in all three panels—values shown are means from three experiments, bars represent s.e.m. ( c ) Densitometry from western blots of fractions from sucrose velocity gradients, comparing the distribution of cavin 1 complexes from control and caveolin 1 −/− lung and heart tissues. Colour key indicates which profile is from each genotype. Values shown are means from three experiments, bars represent s.e.m. Note that the absolute abundance of cavin 1 in caveolin 1 −/− tissues is much less than controls, and all data are normalized to show relative abundance in different fractions, peak fraction=1. Full size image To ascertain whether caveolin 1 has an effect on the different distribution of cavin complexes in the lung and the heart, we analysed these tissues using sucrose velocity gradients from control and caveolin 1 −/− mice and western blotting for cavin 1 ( Fig. 5c ). Comparing caveolin 1 −/− with controls, cavin 1 was still found in large complexes, the distribution of these complexes peaked at approximately the same point in the gradient, and cavin 1-containing complexes still had a clearly different apparent size between the lung and the heart ( Fig. 5c ). Therefore, although there was some decrease in the abundance of cavin 1 in the densest fractions from caveolin 1 −/− samples from both tissues, it is likely that cavin complexes form differently in the heart and the lung independently from caveolin 1. The role of cavin 2 in lung endothelial cells One complication in the interpretation of the sucrose gradient data outlined above is that there is a range of cell types, each potentially with a different complement of cavins and caveolins, in each tissue. To gain further insight into the role of cavin 2 specifically in the lung endothelial cells, where it has an important role in the morphogenesis of caveolae, we established cultures of endothelial cells isolated from the lung of mice with different genotypes. In the cavin 2 −/− cells, there was a reduction in the abundance of caveolae and the residual caveolae were shallower than controls ( Fig. 6a–c ). There was no change in the abundance of caveolae in cavin 3 −/− cells ( Fig. 6b ). Cavin complexes, analysed using sucrose velocity gradients as previously, and detected by blotting of fractions with antibodies against cavins 1 and 3, had a similar size in the cultured control cells as in control lung tissue ( Fig. 6d : compare with Fig. 4b ). Crucially, however, in the cavin 2 −/− cells cavin complexes were significantly larger than in controls, in fact resembling those found in the heart in size ( Fig. 6d : compare with Fig. 4b ). Cavin 1 cofractionated with cavin 3 in both control and cavin 2 −/− cells ( Fig. 6d ), so the increase in size of complexes upon deletion of cavin 2 is likely to represent the behaviour of bona fide cavin complexes rather than aggregation or other aberrant behaviour. Therefore, the changes in abundance and shape of caveolae, and in the apparent size of cavin complexes, in cavin knockout lung endothelial cells recapitulate those observed in the lung in vivo . The data confirm that cavin 2 is indeed responsible for the reduced size of cavin complexes in the lung endothelial cells. 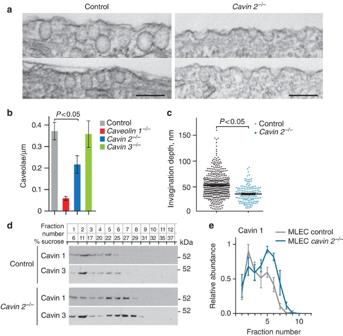Figure 6: Deletion of cavin 2 increases the apparent size of cavin complexes. (a) Electron micrographs comparing the morphology of caveolae from control andcavin 2−/−lung endothelial cells. Note that the abundance of caveolar invaginations in thecavin 2−/−sample is over-represented in these images selected to show examples of typical morphology. Bars, 100 nm. (b) Quantification of the abundance of morphological caveolae in the lung endothelial cells from control,caveolin 1−/−,cavin 2−/−andcavin 3−/−mice.N=12 cells, each reconstructed from 20–30 individual micrographs tracing the cell perimeter. Bars are s.e.m. (c) Quantification of the depth of caveolar membrane invaginations seen incavin 2−/−lung endothelial cells in culture. Depth was measured in electron micrographs as illustrated ina.N>200. (d) Western blots using antibodies against cavins 2 and 3 of fractions from sucrose velocity gradients analysing extracts from control andcavin 2−/−lung endothelial cells. (e) Densitometry showing the distribution of cavin 1 on gradients as ind. Values shown are means from three separate experiments, bars are s.e.m. Figure 6: Deletion of cavin 2 increases the apparent size of cavin complexes. ( a ) Electron micrographs comparing the morphology of caveolae from control and cavin 2 −/− lung endothelial cells. Note that the abundance of caveolar invaginations in the cavin 2 −/− sample is over-represented in these images selected to show examples of typical morphology. Bars, 100 nm. ( b ) Quantification of the abundance of morphological caveolae in the lung endothelial cells from control, caveolin 1 −/− , cavin 2 −/− and cavin 3 −/− mice. N =12 cells, each reconstructed from 20–30 individual micrographs tracing the cell perimeter. Bars are s.e.m. ( c ) Quantification of the depth of caveolar membrane invaginations seen in cavin 2 −/− lung endothelial cells in culture. Depth was measured in electron micrographs as illustrated in a . N >200. ( d ) Western blots using antibodies against cavins 2 and 3 of fractions from sucrose velocity gradients analysing extracts from control and cavin 2 −/− lung endothelial cells. ( e ) Densitometry showing the distribution of cavin 1 on gradients as in d . Values shown are means from three separate experiments, bars are s.e.m. Full size image We used indirect immunofluorescence and confocal microscopy to further characterize the mis-formation of caveolae in cavin 2 −/− lung endothelial cells, by following co-localization between caveolin 1 and cavin 1. In control and cavin 3 −/− cells, caveolin 1 and cavin 1 co-localized in membrane puncta typical of caveolae ( Fig. 7a ). In cavin 1 −/− cells, caveolin 1 staining was weak and diffuse, consistent with the reduced size of caveolin 1 complexes in sucrose gradients ( Fig. 7b ), and previous observations suggesting that caveolin 1 does not form stable oligomers in the absence of cavin 1 (refs 20 , 21 , 43 ). In cavin 2 −/− cells, however, caveolin 1 and cavin 1 co-localized, and could not be distinguished from controls ( Fig. 7a ), and there was no decrease in the size of caveolin 1 complexes in sucrose gradients. In contrast, deletion of cavin 1 caused a pronounced reduction in the size of caveolin 1 complexes ( Fig. 7b ). 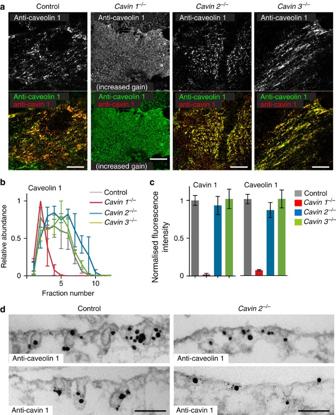Figure 7: Deletion ofcavin 2causes flattening of caveolae without perturbing oligomerization of caveolin 1. (a) Indirect immunofluorescent staining of cultured lung endothelial cells (MLEC) from control,cavin 1−/−,cavin 2−/−andcavin 3−/−mice, using anti-caveolin-1 and anti-cavin-1 antibodies. The top panels show staining for caveolin 1 alone, the lower panels dual colour labelling with both antibodies. Note that there is much less caveolin 1 incavin 1−/−cells than in the other genotypes, and the microscope gain settings were increased when imagingcavin 1−/−cells. Bars, 5 μm. (b) Densitometry from blots of fractions from sucrose velocity gradients analysing the distribution of caveolin 1 in control,cavin 1−/−,cavin 2−/−andcavin 3−/−lung endothelial cells. Note that the absolute abundance of caveolin 1 incavin 1−/−cells is much lower than in other genotypes (seec), data here are normalized so that peak abundance on the gradient=1. Means of three experiments, bars s.e.m., colour key indicates genotype. (c) Quantification of the amount of plasma membrane associated labelling observed with antibodies against caveolin 1 and cavin 1 in the lung endothleial cells with genotypes shown in the key. Images were acquired with total internal reflection illumination to image the basal ~100 nm of cells. Fluorescence intensities were all normalized so that mean from control cells=1, values are mean of >20 cells, bars s.e.m. (d) Pre-embedding immuno-electron microscopy of control andcavin 2−/−cells with caveolin 1 or cavin 1 antibodies. Secondary antibodies were coupled to nano-gold and silver enhancement was used to aid detection of these secondary antibodies. Bars, 100 nm. Figure 7: Deletion of cavin 2 causes flattening of caveolae without perturbing oligomerization of caveolin 1. ( a ) Indirect immunofluorescent staining of cultured lung endothelial cells (MLEC) from control, cavin 1 −/− , cavin 2 −/− and cavin 3 −/− mice, using anti-caveolin-1 and anti-cavin-1 antibodies. The top panels show staining for caveolin 1 alone, the lower panels dual colour labelling with both antibodies. Note that there is much less caveolin 1 in cavin 1 −/− cells than in the other genotypes, and the microscope gain settings were increased when imaging cavin 1 −/− cells. Bars, 5 μm. ( b ) Densitometry from blots of fractions from sucrose velocity gradients analysing the distribution of caveolin 1 in control, cavin 1 −/− , cavin 2 −/− and cavin 3 −/− lung endothelial cells. Note that the absolute abundance of caveolin 1 in cavin 1 −/− cells is much lower than in other genotypes (see c ), data here are normalized so that peak abundance on the gradient=1. Means of three experiments, bars s.e.m., colour key indicates genotype. ( c ) Quantification of the amount of plasma membrane associated labelling observed with antibodies against caveolin 1 and cavin 1 in the lung endothleial cells with genotypes shown in the key. Images were acquired with total internal reflection illumination to image the basal ~100 nm of cells. Fluorescence intensities were all normalized so that mean from control cells=1, values are mean of >20 cells, bars s.e.m. ( d ) Pre-embedding immuno-electron microscopy of control and cavin 2 −/− cells with caveolin 1 or cavin 1 antibodies. Secondary antibodies were coupled to nano-gold and silver enhancement was used to aid detection of these secondary antibodies. Bars, 100 nm. Full size image So as to confirm that there is no change in the amount of caveolin 1 and cavin 1 present at the plasma membrane in cavin 2 −/− cells, the amount of each protein present in total internal reflection images of the basal plasma membrane was quantified ( Fig. 7c ). The amount of caveolin 1 and cavin 1 was the same in control, cavin 2 −/− and cavin 3 −/− cells. As predicted, there was much less caveolin 1 present in cavin 1 −/− cells than in controls ( Fig. 7c ). These findings, coupled with our data showing that the number of morphological caveolae in the cavin 2 −/− cells is around half that observed in controls ( Fig. 6b ), and that the residual caveolae in the cavin 2 −/− cells are significantly shallower than in controls ( Fig. 6c ), implies that a number of the apparently normal caveolin 1/cavin 1 puncta seen by immuno-fluorescence in cavin 2 −/− cells are likely to in fact correspond to flat regions of membrane or aberrantly shallow caveolae. We sought to confirm this inference, using pre-embedding immuno-labelling with caveolin 1 or cavin 1 antibodies and electron microscopy. We could clearly observe the presence of caveolin 1 and cavin 1 in both control caveolae and in the smaller structures seen in cavin 2 −/− cells ( Fig. 7d ). In addition, immuno-EM revealed cavin 1 and caveolin 1 in flat membrane patches in the cavin 2 −/− cells ( Fig. 7d ). These findings demonstrate that cavin 2 is involved in the morphogenesis of caveolar membranes. Deletion of cavin 2 perturbs the lung endothelial morphology The results presented above show that cavin 2 is involved in the formation of caveolae and modulation of cavin complex formation in the endothelium of some tissues, such as the lung, but not others, such as the heart. This predicts that cavin 2 should be required for at least some of the functions of caveolae in lung but not heart endothelium. We examined the ultrastructural morphology of the lung microvascular endothelium, seeking to ascertain whether there are specific changes in caveolin 1 −/− , cavin 1 −/− and cavin 2 −/− animals, where the abundance of caveolae is reduced. In conventional electron micrographs of samples from caveolin 1 −/− cavin 1 −/− and cavin 2 −/− lung we observed, in ~5% of capillary cross-sections, gaps in the normally continuous endothelium ( Fig. 8a ). In the areas containing endothelial gaps neither endothelial cells nor the adjacent epithelial cell layer were well attached to the intervening connective tissue ( Fig. 8a ). Gaps or discontinuities between endothelial cells may represent a more severe consequence of the previously reported reduction in the size of endothelial tight junctions in caveolin 1 −/− lung [36] . The gaps are not an artifact induced by vascular pressure changes during perfusion fixation, as they were also observed in tissue samples fixed without perfusion ( Supplementary Fig. S5 ). In contrast to cavin 2 −/− , c avin 3 −/− lungs were essentially the same as those from congenic controls ( Fig. 8a ), confirming that the phenotype is linked to absence of caveolae and that in the lung cavin 2 −/− pheno-copies cavin 1 −/− and caveolin 1 −/− . 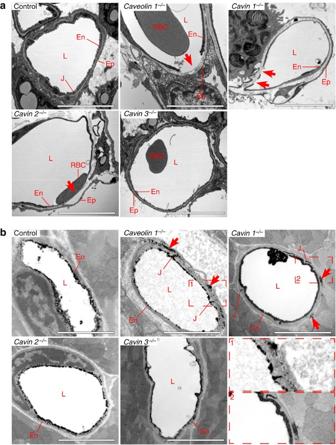Figure 8:cavin 2−/−endothelial morphology resembles that ofcaveolin 1−/−micein the lung but is normal in the heart. (a) Electron micrographs of capillaries from the lung of mice with the genotypes indicated. Red arrows indicate gaps between endothelial cells. L, lumen of capillary; En, endothelial cell; Ep, epithelial cell; J, endothelial tight junction; RBC, red blood cell (not present in all images). Bars, 5 μm. Tissue was taken from 20- to 25-week-old female mice with the genotypes indicated. (b) Perfusion fixation with Lanthanum ions produces electron-dense deposits on cell surfaces accessible from the vascular lumen. Tissue was taken from 20- to 25-week-old female mice with the genotypes indicated. Transverse sections of microvascular capillaries from the heart are shown, lanthanum staining is restricted to the luminal face of blood vessels in all samples exceptcaveolin 1−/−andcavin 1−/−. In these two genotypes lanthanum deposits are observed between cells and outside of the endothelial layer, as showed in the magnified regions indicated with red dashed boxes and highlighted with arrows. Bars, 5 μm. Figure 8: cavin 2 −/− endothelial morphology resembles that of caveolin 1 −/− mice in the lung but is normal in the heart. ( a ) Electron micrographs of capillaries from the lung of mice with the genotypes indicated. Red arrows indicate gaps between endothelial cells. L, lumen of capillary; En, endothelial cell; Ep, epithelial cell; J, endothelial tight junction; RBC, red blood cell (not present in all images). Bars, 5 μm. Tissue was taken from 20- to 25-week-old female mice with the genotypes indicated. ( b ) Perfusion fixation with Lanthanum ions produces electron-dense deposits on cell surfaces accessible from the vascular lumen. Tissue was taken from 20- to 25-week-old female mice with the genotypes indicated. Transverse sections of microvascular capillaries from the heart are shown, lanthanum staining is restricted to the luminal face of blood vessels in all samples except caveolin 1 −/− and cavin 1 −/− . In these two genotypes lanthanum deposits are observed between cells and outside of the endothelial layer, as showed in the magnified regions indicated with red dashed boxes and highlighted with arrows. Bars, 5 μm. Full size image We next examined endothelial morphology in the heart. Conventional electron microscopy did not reveal obvious changes, beyond the presence or absence of caveolae, in any of the genotypes we examined (not shown). As conventional electron microscopy does not report directly on the functional status of tight junctions, we sought a more sensitive electron-microscopy-based assay for altered endothelial permeability. We perfused mice with fixative containing lanthanum ions. Lanthanum forms electron-dense precipitates on polysaccharides present in the glycocalyx, and so perfusion fixation in the presence of lanthanum provides a means of discerning whether the lumen of capillaries is continuous with the extravascular space [44] , [45] . Lanthanum deposits clearly highlighted the capillary luminal face of endothelial cells in the heart ( Fig. 8b ). In the case of caveolin 1 −/− and cavin 1 −/− mice, additional lanthanum deposits were observed in the interstitial space between the endothelium and adjacent cardiomyocytes, providing direct evidence for increased endothelial permeability ( Fig. 8b ). This was not the case in cavin 2 −/− mice, or in controls and cavin 3 −/− . Surprisingly then, in both the lung and heart cavin 3 does not appear to be required for making endothelial caveolae, or for the function of caveolae in terms of maintaining endothelial morphology and hence barrier function. Endothelial phenotypes of cavin 2 −/− mice resemble those of congenic controls in the heart, but those of cavin 1 −/− and caveolin 1 −/− in the lung. This means that cavin 2 is likely to be required for the function of endothelial caveolae in the lung but not in the heart. The identification of the cavin proteins as key components of caveolae with differing tissue distributions [27] suggested the hypothesis that expression of different complements of cavin proteins confers different properties on caveolae in different tissues [17] . The assembly of a set of mouse strains lacking genes for caveolin 1, cavin 1, cavin 2 and cavin 3 has allowed us to test this hypothesis. Three main lines of evidence confirm that endothelial caveolae are heterogeneous between tissues; the differential requirements for cavin 2 expression in caveolar morphogenesis in different endothelia, the variation in the apparent sizes of cavin complexes in different tissues and the differential functional consequences of deletion of cavin 2 in terms of altered endothelial morphology. Our data reveal that cavin 2 is required for generating caveolae in some types of endothelium but not others, and that cavin 3 is dispensable for formation of endothelial caveolae. Therefore, in some contexts, but not in others, cavin 1 and caveolin 1 may be sufficient for generating caveolae [27] . We speculate that the explanation for this apparent paradox lies in the different nature of the complexes into which cavins can assemble. In tissues where cavin 2 is needed for making caveolae, cavin 1 runs on sucrose gradients as much smaller complexes than in other tissues. It is possible that this reduced apparent size in fact represents reduced stability of complexes during extraction and analysis, rather than differences in the size of cavin complexes in situ . In either eventuality, however, the conclusion that the properties of cavin complexes are different in different tissues remains valid. Information on the structure of different cavin complexes, how assembly of the complexes is controlled, and whether further tissue-specific components are present, is lacking. It is also possible that association of further, non-cavin, proteins could directly influence the size of cavin complexes. Despite the uncertainties outlined above, the data do provide clear evidence that the cavin proteins have quite different roles. Cavin 1 is required to mediate or maintain the normal oligomerization of caveolin 1 (refs 18 , 20 , 21 ), and our experiments reveal that cavin 1 co-localizes with oligomerized caveolin 1 in cells that lack cavin 2 even when this does not result in formation of morphological caveolae with normal efficiency, as is the case in the lung endothelial cells. Cavin 2 is, therefore, required for caveolar morphogenesis in specific contexts. Consistent with our findings in cultured lung endothelial cells lacking cavin 2 , flattened or shallow caveolae are observed in cavin 2 short hairpin RNA-treated adipocytes [33] . Unlike cavin 1, cavin 2 does not directly stabilize caveolin 1 oligomers. Rather, cavin 2 has a strong effect on formation of cavin complexes, the presence of cavin 2 reducing the size or stability of these complexes. Although the cavin proteins do clearly form a single protein family [17] , our data argue that they are not functionally interchangeable. There is no detectable expression of cavin 4 in endothelial cells when cavin 2 or cavin 3 are deleted, so cavin 4 is unlikely to compensate for the lack of other cavins in endothelial cells. Even in the case of cavin 3 in cavin 2 −/− animals, where there is some upregulation of protein expression, our data on the quantification of caveolar abundance in cavin 2 −/− cavin 3 −/− double knockout animals implies that cavin 3 does not compensate, in this respect at least, for the lack of cavin 2 . It is possible that specific aspects of caveolar function are dependent on expression of cavin 3. Intriguingly, these functions would then probably not require the characteristic morphology of caveolae. None of our observations using electron microscopy report the complete absence of caveolae. This is at least in part likely to be because we have relied on a purely morphological definition of caveolae, and flask-shaped invaginations of the plasma membrane may be generated in several ways—for example, a vesicle in the process of fusion with the plasma membrane could be ultrastructurally very similar to caveolin-positive caveolae. It also remains possible that there is an alternative mechanism for generating caveolae [46] . Previous studies on the role of cavin 2 in generating caveolae report slightly more severe loss of caveolae, as well as reduced expression of caveolin 1, in cultured adipocytes or HeLa cells following short hairpin RNA-mediated knockdown than we observe in vivo [18] , [27] , [33] . The reason for this is unclear, but potential explanations include differences between cell type and the possibility that partial loss of cavin 2 causes different effects from complete loss of the protein. Cardiovascular phenotypes in mutant animals lacking caveolae indicate a role in endothelial permeability [3] , [11] , [35] , [36] . These phenotypes are likely to be due to functions for caveolae as transcytotic vesicles [10] , as regulators of eNOS activity [3] , and as sensors of mechanical stress [2] , [47] , [48] . Our data showing that endothelial caveolae differ biochemically and are generated in different ways between tissues suggest a mechanism by which alternative aspects of caveolar function may be carried out by these morphologically quite uniform structures. The endothelium of different tissues is highly heterogeneous in terms of both morphology and function [7] , [49] , [50] , and cavin 2 is one of the molecular components that generates this heterogeneity. Mouse genetics and husbandry To produce cavin 2 or cavin 3 gene knockout mice, targeted embryonic stem cells (clone names 11065A-H7 and 11448A-D8, respectively) generated by the trans-NIH Knock-Out Mouse Project (KOMP) were obtained from the KOMP Repository ( www.komp.org ). The ES cells were injected into separate blastocysts derived from C57BL6 mice and implanted into pseudo-pregnant females using standard techniques. Resulting heterozygous+/− chimeric animals were backcrossed to C57Bl/6. Cavin 1 (PTRF) knockout animals were obtained from the Jackson Laboratories ( www.jax.org ) and have previously been described [28] . Likewise, caveolin 1 knockout animals [30] were obtained from the Jackson Laboratories and backcrossed onto C57Bl/6 background for seven generations. Loss of the genomic locus of interest was confirmed by PCR ( Supplementary Fig. S1 ). Genotyping was carried out by a multiplex PCR, primers used are shown in Supplementary Table S1 . Changes in gene expression were confirmed by quantitative PCR (lack of messenger RNA, not shown) and western blotting ( Fig. 1 and Supplementary Fig. S2 ). Mice used in all experiments were sex and age matched, kept in individually ventilated cages in pathogen-free conditions and fed a standard chow (from Special Diets Services). All animal experiments were undertaken with the approval of the UK Home Office and local MRC-LMB Ethical Review Committee. DNA constructs and antibodies All DNA constructs have been described previously [18] , [41] . Sources for antibodies were as follows: rabbit polyclonal anti-PTRF (Cavin1) (ab48824), rabbit polyclonal anti-PRKCDBP (Cavin3) (ab83913), rabbit polyclonal anti-Caveolin3 (ab2912) and goat polyclonal anti-EHD2 (ab23935) were all from Abcam. Polyclonal rabbit anti-caveolin 1 (Ab 610059) and mouse monoclonal anti caveolin 2 (Ab 610685) were both from BD Biosciences). Monoclonal antibodies raised against caveolin 1 were generously provided by Jørgen Vinten (The Panum Institute, University of Copenhagen, Denmark) [51] . Polyclonal Goat anti SDPR (Cavin2) is raised against the N-terminal part of the protein. Polyclonal Rabbit anti SDPR (Cavin2) is raised against the C-terminal part of the protein. Polyclonal rabbit anti-MURC (Cavin4) is raised against the C-terminal part of the protein. HRP-conjugated secondary antibodies were from DAKO and the ECL western blotting detection kit was from GE Healthcare. Light microscopy Mice were culled by cervical dislocation, tissues were dissected and immediately frozen on dry ice and stored at −80 °C until processed. Frozen sections were cut on a microtome (Leica CM3050S). Sections were transferred onto frosted microscope slides (Thermo Scientific) and air dried for 2 h, fixed in 4% paraformaldehyde (PFA) in PBS for 1 h, washed, labelled with the appropriate antibodies, and finally overlaid with 4',6-diamidino-2-phenylindole Fluoromount-G (SouthernBiotech). Images were acquired with a Plan-Apochromat 40 × 1.3oil DIC M27 objective on a Zeiss 780 confocal microscope with standard filter settings. The gamma was increased in red/green overlay images to allow visualization of co-localization. Electron microscopy Perfusion fixation of mice was carried out under anaesthesia, via injection into the left ventricle and cutting of the right atrial chamber. Blood was flushed away using an initial perfusate of Hanks buffered salt solution+heparin. Standard transmission electron microscopy Tissues were then perfused with fixative containing 2.0% PFA, 2.5% glutaraldehyde (GA) in 0.1 M sodium cacodylate buffer pH 7.4. The heart, liver, kidney, fat, lung and abdominal muscle were then rapidly dissected and placed in fresh fixative. The same protocol was followed for tissues fixed without perfusion, except that the initial fixative was supplemented with 4 mM CaCl 2 . Following several buffer washes, tissues were post fixed in 1% osmium tetroxide in 0.1 M sodium cacodylate buffer for 1 h at 4 °C. Tissues were then enbloc stained with 2% uranyl acetate in 30% ethanol and further dehydrated in an increasing ethanol series, followed by propylene oxide and infiltration and embedding in CY212 resin. Sections were counterstained with Reynolds Lead Citrate and viewed on a Philips 208 microscope operated at 80 kV. Quantification of caveolae in endothelium was carried out as described previously [18] . Lanthanum tracer studies Following perfusion with Hanks buffered salt solution+heparin, mice were perfused with fixative containing lanthanum chloride (3.0% PFA, 2.5% GA and 1% lanthanum chloride in 0.1 M pipes buffer pH 7.2 at room temperature (RT) for 15 min, followed by the same fixative minus the LaCl for several hours. Tissue specimens were then washed in 0.1 M pipes buffer, and then post-fixed in 1% osmium tetroxide in 0.1 M sodium cacodylate for 1 h on ice, enbloc stained with 7% uranyl acetate in water for 2 h at 4 °C, and dehydrated and processed as for as above. Immuno-labelling Endothelial cells were grown on gelatine-coated glass bottom Petri dishes (MatTek) and fixed in 4% PFA in 0.1 M phosphate buffer pH 7.4 overnight at 4 °C. After several buffer washes, followed by inactivation of reactive aldehyde groups using 0.1% sodium borohydride in phosphate buffer for 15 mins, cells were permeabilized using 0.03% saponin in 20 mM phosphate buffer, 150 mM sodium chloride for 30 mins. Cells were incubated in normal goat serum (Aurion) for 40 min before incubation in rabbit anti-caveolin 1 antibody used at 1:200 for 4.5 h at RT. After thorough washing, cells were incubated with 1:200 dilution of goat anti rabbit ultrasmall gold (Aurion) overnight at 4 °C. After washing cells were fixed with 2% GA in 0.1 M phosphate buffer for 30 min, washed with distilled water followed by silver enhancement of gold using R-Gent SE-EM (Aurion) reagents. Cells were then post fixed with 0.5% osmium tetroxide in 0.1 M phosphate buffer on ice for 15 mins. Cells were then dehydrated in an ascending ethanol series and embedded in CY212 resin. Ultrathin sections were stained with saturated aqueous uranyl acetate and Reynolds lead citrate and examined using a Philips 208 EM operated at 80 kV. Sucrose velocity gradients We used a protocol based on that of Hayer et al . [43] Different tissues were washed in PBS and approximately 0.05 g of tissue was homogenized using a Dounce homogenizer in 1 ml of 0.5% Triton X100 in 100 mM NaCl, 20 mM Tris–HCl pH 7.4, 5 mM EDTA, supplemented with ‘Complete’ protease inhibitors (Roche). The samples were next incubated in RT for 20 min. Post-nuclear supernatant (PNS) was prepared by a 6-min centrifugation at 1,100 g . 800 μl of PNS was loaded onto step gradient of 40, 35, 30, 25, 20 and 10% sucrose containing 0.5% TX100, 20 mM Tris–HCl pH 7.4, 100 mM NaCl, 5 mM EDTA and protease inhibitors. For analysis of extracts from endothelial cells, one Petri dish containing cells was solubilized in 1 ml 0.5% TX100, 20 mM Tris–HCl pH 8, 300 mM NaCl, 5 mM EDTA. PNS was loaded onto a step gradient of 40, 35, 30, 25, 20 and 10% sucrose containing 0.5% TX100, 20 mM Tris–HCl pH 8, 300 mM NaCl, 5 mM EDTA. The gradients were centrifuged at 4 ˚C in SW40 rotor (Beckman) for 270 min at 245,000 g with slow acceleration and deceleration. Twelve 900 μl fractions were collected from the top of the gradient, and densities of the fractions were calculated from the refractive indices. From each fraction, 200 μl samples were precipitated using 10% trichloroacetic acid and pellets were analysed by SDS—polyacrylamide gel electrophoresis/western blot. Purified ribosomal samples for calibration were a kind gift from Alexey Amunts (MRC-LMB). Western blotting Mice were culled by cervical dislocation, tissues were removed and immediately frozen on dry ice and either processed the same day or stored at −80 °C. Tissues were homogenized with an IKA-Werke homogenizer in 0.5 ml RIPA buffer supplemented with protease inhibitor tablets (Roche). The homogenized tissues were left rolling at 4 °C for 3 h, and the homogenate was cleared by centrifugation at 16,000 g for 10 min. The supernatant, or samples from fractionation as described above, were mixed with reducing sample buffer, boiled and run on pre-cast 4–20% Tris-glycine gels (Invitrogen). The gels were blotted using a semi-dry blotter (Bio-Rad) and the membrane blocked in a PBS solution containing 4% dried skimmed milk powder and incubated with the appropriate antibodies, washed and incubated with secondary antibodies (DAKO). The blots were developed using Immobilon (Millipore) onto Fuji Super RX X-ray films. Endothelial cell culture Mice were killed by cervical dislocation, lungs dissected, finely chopped with a scalpel blade and digested in collagenase for 2 h. The cell mixture was run through a 70-μm nylon cell strainer (BD Falcon), spun down and suspended in mixed medium (50% low-glucose DMEM (Gibco), 50% F12 Nut Mix (Gibco) supplemented with 20% FCS and 100 μg ml −1 endothelial cell mitogen (Serotec). The cell mixture was then seeded onto one 0.1% gelatin-coated chamber (Sigma) of a six-well plate per lung equivalent. The medium was changed the following day. After 4–6 days in culture the cells were trypsinized and endothelial cells were immuno-isolated using rat anti-mouse CD102 antibodies (BD Pharmigen) and dynabeads (Dynal Biotech). Isolated endothelial cells were hereafter plated on 0.1% gelatin-coated plastic. Endothelial cell purity was assessed by morphology at confluency, and positive expression of VE-Cadherin. How to cite this article: Hansen, C. G. et al . Deletion of cavin genes reveals tissue-specific mechanisms for morphogenesis of endothelial caveolae. Nat. Commun. 4:1831 doi: 10.1038/ncomms2808 (2013).